Forensic genomics as a novel tool for identifying the causes of mass mortality events Toxic spills, hypoxia, disease outbreaks and toxin-producing algal blooms are all possible causes of mass mortality events, but in many cases it can be difficult to pinpoint the cause of death. Here we present a new approach that we name ‘forensic genomics’, combining field surveys, toxin testing and genomic scans. Forensic genomics queries allele frequencies of surviving animals for signatures of agents causing mass mortality and, where genetic diversity is high, is uniquely suited to identify natural selection in action. As a proof of concept, we use this approach to investigate the causes of an invertebrate mass mortality event, and its genetic effects on an abalone population. Our results support that a harmful algal bloom producing a yessotoxin was a major causative agent to the event. Mass mortality events have been reported throughout the animal kingdom [1] , [2] , [3] , [4] , [5] , and in many cases it is difficult to pinpoint the agent responsible. One major cause of recent marine mortality events are harmful algal blooms (HABs) [3] , [6] , [7] , [8] that kill either by toxin production or by hypoxia caused by decomposing algae [8] . Toxin-induced mortality is often difficult to identify since putatively causal toxins must be individually tested for levels and toxic effects in most cases [9] , [10] , as simultaneous screening of multiple toxins requires a significant infrastructure [11] . If the toxin is novel, toxicity data or presence/absence tests may be non-existent, making it difficult to infer mortality causation. However, it is possible that the surviving population may harbour a distinct genomic signature of toxin-induced natural selection, which would manifest as genetic variants (single nucleotide polymorphisms; SNPs) with abnormally high F ST values in before–after comparisons [12] . In addition, gene functions related to the cause of mortality might be enriched in high F ST SNPs. In many cases, there is some knowledge of the cellular targets of classes of potential toxins [13] , [14] , so by matching genomic data with what is known about putative causal toxins, it would in theory be possible to test hypotheses about the potential causes of a mortality event. As a demonstration of this novel method, we examined a 2011 algal bloom-associated mass mortality event of a marine gastropod, the red abalone, Haliotis rufescens , in California [15] . This was a unique event, being the largest invertebrate die-off ever recorded in the region. Crabs, sea urchins and abalone were all affected simultaneously and showed high mortalities, whereas other taxa such as bat stars were not, suggesting an external mortality agent rather than a wholesale collapse of environmental quality such as hypoxia. Toxin testing was inconclusive, but suggested that a member of the yessotoxin (YTX) family could potentially be involved. YTX has a well-characterized mode of action affecting cytoskeleton organization (especially cadherin) [14] , [16] , [17] , the apoptosis pathway [18] , [19] , [20] , electron transport chain proteins [19] , [21] and the immune system [22] . We hypothesized that YTX effects on abalone would manifest in SNP frequency changes at some of these pathways, whereas metabolic pathways of other classes of toxins would remain unchanged. For example, unlike common HAB toxins, such as microcystins or okadaic acid and its derivatives, YTXs do not inhibit protein phosphatases [23] , so if any of the above toxins were the cause of the mortality event, we would expect to see changes in protein phosphatases in before–after comparisons [23] , [24] . If hypoxia contributed to the mortality, we would also see changes in genes known to confer hypoxia tolerance (such as HIF-1a and arginine kinase ) [25] , [26] as well as enrichment for high F ST SNPs in the gene ontogeny (GO) functional category ‘response to hypoxia’. In addition, as YTX is an organic cyclic compound [24] , [27] , we would expect the GO functional category ‘response to organic cyclic compound’ to be enriched for high F ST SNPs if YTX was the cause. These hypotheses depend on the existence of standing genetic variation for response to YTX in abalone. However, the high levels of genetic polymorphism in abalone [25] together with the potentially adaptive role of genetic diversity in loci involved in toxin tolerance in the natural environment suggest that this type of variation may exist. In addition, recent work showing that high-diversity invertebrates have genetic responses to other environmental stressors such as heat [28] and acidification [29] suggest that this might also be the case for toxin tolerance. Although multiple causes cannot be ruled out, the genomic data support YTX being involved in the mass mortality event, through the effect of YTX on mitochondrial function and cadherin binding. Our data also implicate a well-known detoxification gene [30] , glutathione-S-transferase , in abalone toxin tolerance. Our results suggest that red abalones have genetic variation for response to YTX effects particularly in alleles at cadherin loci. Field surveys indicate high mortality Field surveys at four different sites ( Fig. 1 ) were conducted before and after the HAB event, which occurred at the end of August 2011. Mortalities ranged from 20 to 44.5% when averaged across three-depth zones (mean 25%), with the highest mortalities in shallow depth (<5 m, mean 48%, s.e. 13.5) ( Fig. 2 ). Abalone densities dropped markedly at all four sites during the event and have remained low until present, prompting the California Fish and Game Commission to reduce the yearly take limit state-wide and to close the Fort Ross site completely in June 2013. Abalones in flow-through, oxygenated aquaria at a nearby marine laboratory were also killed, suggesting that hypoxia was not the cause of the event [15] . Known abalone diseases such as ‘Withering-foot syndrome [31] were ruled out because dead animals lacked characteristic withering symptoms of the disease. 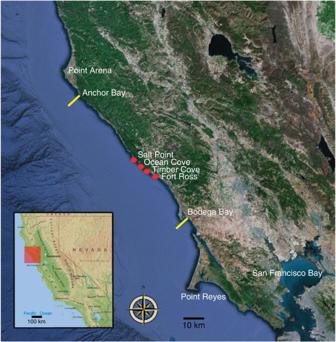Figure 1: Map of Sonoma County, California. The geographical extent of the mortality event (marked with yellow lines) from Anchor Bay in the north to Bodega Bay in the south, as well as field survey locations indicated by red circles. Figure 1: Map of Sonoma County, California. The geographical extent of the mortality event (marked with yellow lines) from Anchor Bay in the north to Bodega Bay in the south, as well as field survey locations indicated by red circles. 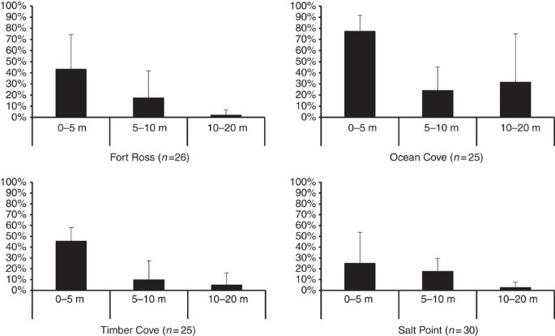Figure 2: Red abalone mortality by depth. Mean transect percent mortality of red abalone along 30 × 2 m2transects at the four survey sites in Sonoma County with s.d. error bars (abalone tissue samples for genomic work were taken from 0–5 m depth at Fort Ross). Full size image Figure 2: Red abalone mortality by depth. Mean transect percent mortality of red abalone along 30 × 2 m 2 transects at the four survey sites in Sonoma County with s.d. error bars (abalone tissue samples for genomic work were taken from 0–5 m depth at Fort Ross). Full size image Toxin testing inconclusive Reports of an algal bloom in coastal waters during this time suggested that an algal-produced toxin might be responsible [15] . To test this, mussels, abalone and sea stars were tested for a wide range of known HAB toxins, including anatoxin-a, azaspiracids 1–5, domoic acid, lyngbyatoxin, microcystins, okadaic acid, saxitoxins, YTX and homo-YTX, with all but one showing no detectable levels ( Supplementary Data 1 ). The exception was one class of algal toxins, YTX (maximum concentration 999 ng g −1 ), which was detected in the digestive glands of sickly abalone from Fort Ross. Additional testing found lower levels of YTX (15–559 ng g −1 ; n =15) in mussels and abalone digestive glands collected at Bodega Head, North Timber Cove, Potato Patch and Fort Ross. YTXs comprise a large family of toxins: at least 90 varieties of YTX have been isolated from a variety of phytoplankton and shellfish taxa [32] . Four variants are regulated in shellfish for human consumption by the European Union with a limit of 1,000 ng g −1 YTX [27] . However, nothing is known of YTX critical concentrations in invertebrates, and previous testing has shown YTX to be present up to 60 ng g −1 in non-bloom, non-mortality conditions [33] . Forensic genomics implies Yessotoxin as cause of mortality Previous to the die-off, we had surveyed the transcriptome of this abalone population for SNP markers [25] . The population has high genetic diversity and shows strong patterns of evolutionary response to local environmental conditions such as upwelling and acidification [25] . After the die-off, we were able to resample the population and compare transcriptomic-wide SNP frequencies pre- and post-mortality for signatures of natural selection at 15,016 loci. Using an F ST outlier approach, we found 222 SNPs that were more divergent than expected under neutrality. Of these, 42 SNPs are within 34 annotated genes, which were more divergent than expected under neutrality ( Fig. 3 , Table 1 , Supplementary Data 2 ), including genes related to cytoskeleton organization, electron transport chain, protein folding and response to organic cyclic compounds ( Fig. 4 , Supplementary Data 3 ) (high F ST gene ontology over-representation analysis, Benjamini–Hochberg adjusted P -value <<0.001, n SNPs =27,610). Out of these, Se-cadherin ( F ST =0.215) shows a particularly strong series of changes. YTX is known to target cadherin [14] , [17] , causing a cascading effect of cytoskeleton disruption. In the Cadherin gene, the outlier SNP is located in the cytoplasmic region of the protein (pfam01049), responsible for catenin binding [14] . The outlier does not code for an amino-acid change. However, it is linked to a series of SNPs of unknown function in the 3′UTR, as well as to a series of silent SNPs up to 2,000 bp upstream that increased in frequency by 65% during the die-off ( Fig. 5 ). The functional role of these changes is not known. 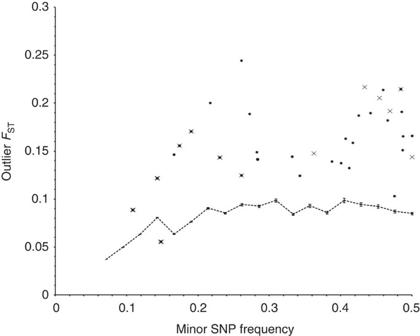Figure 3: OutlierFSTplotted against minor allele frequency. Plot of outlier SNP minor variant frequency versusFST,comparing mean outlierFSTbetween randomly permuted populations from the original dataset (dotted line,nREPLICATES=100, error bars are 95% confidence intervals) and SNP outliers in the actual before–after comparison (dots and crosses; the crosses represent well-annotated SNPs, the remainder are marked as dots). Figure 3: Outlier F ST plotted against minor allele frequency. Plot of outlier SNP minor variant frequency versus F ST, comparing mean outlier F ST between randomly permuted populations from the original dataset (dotted line, n REPLICATES =100, error bars are 95% confidence intervals) and SNP outliers in the actual before–after comparison (dots and crosses; the crosses represent well-annotated SNPs, the remainder are marked as dots). Full size image Table 1 Outlier genes. 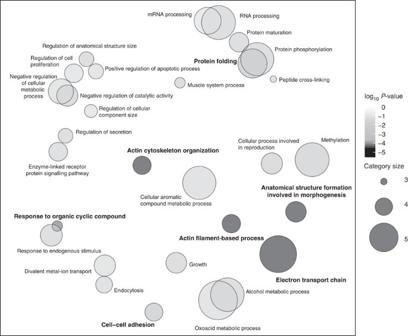Figure 4: Gene functions enriched for highFST. ReVIGO scatterplot of GO categories enriched for highFSTSNPs (GO over-representation analysis (ORA), Benjamini–Hochberg correctedP<0.05,nSNPs=27,610), with darker circles denoting higher enrichment, circle size denoting breadth of the GO category and semantically similar (simRel) GO terms closer to each other (highly enriched (P<10−3) categories are marked in bold font). Full size table Figure 4: Gene functions enriched for high F ST . ReVIGO scatterplot of GO categories enriched for high F ST SNPs (GO over-representation analysis (ORA), Benjamini–Hochberg corrected P <0.05, n SNPs =27,610), with darker circles denoting higher enrichment, circle size denoting breadth of the GO category and semantically similar (simRel) GO terms closer to each other (highly enriched ( P <10 −3 ) categories are marked in bold font). 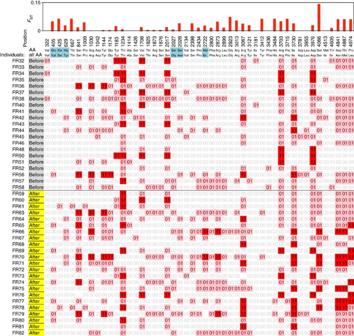Figure 5: Cadherin SNP map. Map of SNPs, genotypes andFSTalong the Cadherin contig (contig14782) in red abalone in Sonoma pre- and post-mortality, not including singletons and SNPs located in the UTR (amino-acid replacements are highlighted in blue). Full size image Figure 5: Cadherin SNP map. Map of SNPs, genotypes and F ST along the Cadherin contig (contig14782) in red abalone in Sonoma pre- and post-mortality, not including singletons and SNPs located in the UTR (amino-acid replacements are highlighted in blue). Full size image Our data also show a multitude of cytoskeletal genes and functional categories related to cytoskeletal organization with outlier SNPs. In addition, cellular homeostasis and divalent metal-ion transport ( P =0.03), as well as regulation of programmed cell death and apoptosis ( P =0.03) are enriched for high F ST SNPs. Another target seems to be mitochondrial function [19] , [21] , for which alleles at fructose-biphosphate aldolase (3 outliers with F ST >0.1) seem to be especially related to toxin survivability. It is known that changes in intracellular calcium homeostasis disrupt mitochondrial membrane potential, inhibiting the electron transport chain [24] . Furthermore, glutathione-S-transferase , known in insects [30] to be involved in detoxification of a wide range of exogenous compounds, contains three high F ST SNPs, and may thus be a potential player in toxin detoxification in abalone. We also examined alternative hypotheses regarding the metabolic pathways that may have been related to the die-off. The GO functional category ‘response to hypoxia’ was not enriched for high F ST SNPs. Genes known to be involved in hypoxia tolerance (for example, HIF-1a (contig88699: n SNPs =27, Max F ST =0.030), arginine kinase (contig90217: n SNPs =15, Max F ST =0.033)) were not affected by the event as indicated by the F ST outlier analysis. SNPs in protein phosphatase-coding sequences ( N =67 across 17 sequences) were not affected by the mass mortality. Because there were no detectable levels of other toxins, such as azaspiracids, saxitoxin, domoic acid, okadaic acid, microcystins, lyngbyatoxin and anatoxin-a, these were effectively ruled out as the drivers of the mortality event. The methods used in this study, combining field studies, toxin testing and genetic forensics, can be used not only to determine the cause of death but also to enhance our understanding of the mechanisms of action at the organismal level. In this case, we can show that the population genomic effects of the mass mortality event are consistent with YTX being a major causative agent, while the combination of toxin testing and genetic sampling could rule out most other HAB toxins as well as hypoxia as main causes (although other factors could have certainly contributed to the event). This method currently depends on the existence of transcriptome-ready samples before a mortality event, a requirement which may not be met in most cases. However, as DNA-based methods of whole-genome analysis at the population level become more affordable, it may be possible to base before–after comparisons on DNA samples from museums or from population genetic monitoring programs. Out of 222 detected F ST outliers, only 42 could be reliably annotated, leaving 180 SNPs with unknown function being affected by the event. These might be contaminants or artifacts of an imperfect assembly, but they might also be of biological importance. As a consequence, we cannot completely rule out additional stressors as contributing to the event. However, as almost all annotated outliers are consistent with YTX as a cause, we can still conclude that the major causative agent was the toxin. It is still unclear why mortalities were greater in shallow waters. It could potentially be due to higher toxin concentrations near the coast [34] , or from wave action increasing the solubility of the toxin. The reduction in mortality at depth is consistent with YTX as a causative agent, as the toxin may have been more concentrated (that is, at toxic concentrations) in shallow depths due to lower water volume and reduced mixing. However, it is important to note that very little is known about the mechanism of action of YTXs, making it difficult to draw specific conclusions about this. Another group of toxins that have similar effects to YTXs is azaspiracids. However, none of the organisms known to produce these toxins ( Azadinium spp. ) were present in the water at the time, and analysis of tissue samples for azaspiracids 1–5 was negative. The presence of two varieties of YTX, confirmed through testing, makes this the prime candidate of the mortality event. In theory [35] , [36] , [37] , a reduction in genetic diversity and an increase in linkage disequilibrium can be seen around selected regions. Unfortunately, we do not know enough about linked regions in the abalone transcriptome. Within single contigs, it is possible to study linkage effects; within the Se-cadherin contig, for example, there are distinct blocks of linked loci visible ( Fig. 5 ). However, without prior knowledge of linkage in the red abalone population, it is hard to draw general conclusions about the selective effects on linkage properties. The outlier analysis suggests a few loci with relatively high F ST values increasing during the event from very low allele frequencies, estimated at 0 (denoted with asterisks in Table 1 ). Although it might be possible that these were present in low frequencies before the event and were selected for, uncertainty in the allele frequency estimation might also account for this pattern. Our sample size of 21–23 per population, while suggested to be adequate for decent allele frequency estimation [38] , might still be too low for low-frequency alleles. Therefore, we have chosen not to focus on these outliers. By gaining insight into the ultimate targets of toxins, and the allelic basis of resistance to them, it may be possible to better identify more resistant natural populations. Such resilience mapping has recently been initiated for coral heat resistance [28] and sea urchin acidification resistance [29] . One management strategy is to protect resilient populations from other sources of mortality, such as habitat destruction or fishing mortality for which they have no resistance. These protected populations may then be able to provide sustained population growth under future climate change scenarios, or contribute to a more productive aquaculture brood stock. Finally, we would urge any future comprehensive ecosystem monitoring programme to include routine acquisition of genetic libraries. The enhanced genetic knowledge gained before a mortality event occurs provides the genetic baseline, which can be compared with the genetics of the population post mortality thereby aiding in identification of the causative agent, as has been done in this example. We suggest that obtaining genetic baseline data is an important part of baseline monitoring of healthy wild populations. Mortality field surveys In September and October 2011 after the mass mortality of marine invertebrates was observed in Sonoma County, a series of three subtidal SCUBA surveys were conducted. Surveys were based at important red abalone fishing grounds within Sonoma County from south to north at Fort Ross (38° 30.1′ N, 123° 13.8′ W), Timber Cove (38° 31.8′ N, 123° 16.4′ W), Ocean Cove (38° 33.1′N, 123° 18.4′ W) and Salt Point (38° 33.7′ N, 123° 19.5′ W) ( Fig. 1 ). Surveys were conducted by experienced subtidal research teams that counted live and dead marine invertebrates along 30 × 2 m 2 transects at three-depth strata (0–5, 5.1–10 and 10.1–20 m) per site. Dead invertebrates were clearly differentiated from live as abalone being unattached to the substrate, upside down with an opaque white foot muscle tissue. Dead sea urchins were not attached to the substrate with spines fallen off the test and dead sea stars had curled-up arms with a white dead colouration to the flesh. The percent of dead invertebrates at each depth and site were recorded. Toxin testing A total of 40 tissue samples were collected between 27 August and 14 September 2011 from the Fort Ross area, Salt Point, Bodega Head, Bodega Harbor, North Timber Cove and Potato Patch ( Supplementary Data 1 ). Samples were shipped frozen to UC Santa Cruz and were kept at −80 °C until processing. Approximately 1 g for each of 32 tissue samples was homogenized with 100% methanol (MeOH), which was subsequently diluted to 50% before cleanup. Samples were then split for toxin analysis of domoic acid, microcystins LR, RR, YR and LA, okadaic acid, saxitoxins, lyngbyatoxin, YTX and homo-YTX. Methanol extracts stored (−20 °C) were also subsequently tested for azaspiracids and re-tested for YTXs. Methodological details for toxins other than YTXs are not reported in detail since samples were negative for all other toxins; these analyses followed standard protocols [39] , [40] using LC–MS for all but saxitoxins, which were screened using commercial enzyme-linked immunosorbent assay kits. Samples for YTX and homo-YTX were initially screened by following the method of Paz et al . [41] with the following modifications. Homogenate (5 ml, 0.5 g tissue) was loaded onto BakerBond C18 cartridges and eluted in 90% MeOH. Samples were analysed on an Agilent 6130 liquid chromatography–mass spectrometry (LC–MS) system with an Agilent Poroshell 120 SB-C18 2.7-μm (2.1 × 50 mm 2 ) column with electro-spray ionization in negative mode [41] . Selected ion monitoring of parent and daughter ions for YTX and homo-YTX was quantified with concentrations determined by comparison with standard curves for YTX and homo-YTX using certified standards (NRC, Canada). From the initial screening, 12 samples were selected for further analysis representing potentially positive and negative samples from mussels, abalone (gill, digestive gland/gonad, foot) and sea star (gonad tissue from the arm). The LC–MS method was adapted to the protocol by These et al . [42] and the tissue samples were hydrolysed [42] . This provided better separation and a lower limit of detection than the initial screening, with a limit of detection for total toxins of 20 ng g −1 tissue (calculated as 3.3 × s.d./ S , where s.d. is the standard deviation and S is the slope of the calibration curve). Archived extracts were subsequently analysed using the same method, but without the hydrolyzation step, for all samples. The method detection limit for these samples was slightly lower than for the hydrolysed samples, at 15 ng g −1 tissue. Hydrolysed samples ( n =4) were of 8–83% higher concentration than non-hydrolysed samples. For reporting purposes, homo-YTX and YTX were summed as total YTX. We did not screen for 45-hydroxy-YTX or 45-hydroxy-homo-YTX (the other two compounds regulated by the European Union). These have toxic equivalence factors of 1.0 and 0.5, so our results are potentially conservative estimates of total toxicity. DNA sequencing and bioinformatics Mantle tissue samples were collected from 24 live red abalone before the bloom (22 April 2011) and 24 abalone after the bloom (17 October 2011) at shallow depths in Fort Ross State Park, Sonoma County, California (38° 30.1′ N, 123° 13.8′ W) ( Fig. 1 ). Total RNA was extracted and cDNA libraries were created from poly-A-selected mRNA. All samples were tagged with barcoded adaptor sequences and sequenced, six individuals per lane in an Illumina HiSeq 2000, for a total of eight lanes. One sample from before the event and one from after the event produced low-read counts, leaving 23 from before and 23 from after for further analysis. Using the protocol of De Wit et al . [43] , reads were filtered from low-quality base calls and residual adaptor sequences, and were then aligned using Burrows-Wheeler Aligner (BWA) [44] to a recently published red abalone mantle transcriptome [25] . SNP detection using GATK [45] resulted in 1,434,378 high-quality ( P >0.99) SNP calls, out of which 46,063 had high-quality genotypes ( P >0.99) for all individuals. A principal components analysis ( Fig. 6a ) showed that two individuals from before the event were significantly (10 −65 ) different from all others in Principal Component (PC) one. Further investigation found that these individuals (FR 39, FR49) were heterozygous at all of the top 500 scoring loci in the PCA, raising the possibility of them being hybrids between red abalone and another co-occurring abalone species. These individuals were removed from the dataset and the SNP detection was rerun, resulting in 1,405,746 high-quality SNPs, out of which 45,966 had high-quality genotypes at all loci. A principal components analysis ( Fig. 6b ) indicated that there was no overall divergence between the before and after populations. 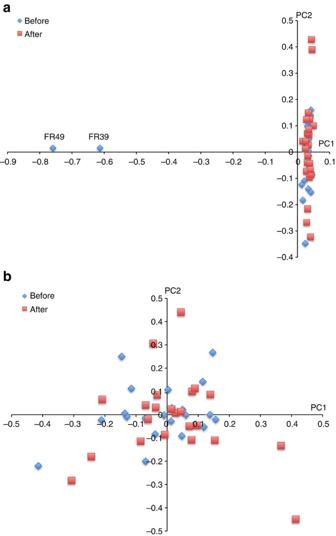Figure 6: Principal components analysis of pre- and post-mortality genetic data. (a) Principal components analysis (PCA) of red abalone individuals before and after the die-off, indicating that individuals FR39 and FR49 were genetically distinct from remaining individuals; they were thus omitted from further analyses. (b) PCA of the same data, after removing individuals FR39 and FR49. Figure 6: Principal components analysis of pre- and post-mortality genetic data. ( a ) Principal components analysis (PCA) of red abalone individuals before and after the die-off, indicating that individuals FR39 and FR49 were genetically distinct from remaining individuals; they were thus omitted from further analyses. ( b ) PCA of the same data, after removing individuals FR39 and FR49. Full size image An F ST outlier analysis was conducted using Lositan Selection Workbench [46] after removing SNP loci obviously out of Hardy–Weinberg equilibrium and loci with low minor allele frequencies (<5%) ( n =15,016). SNPs located above the 95% confidence interval of the overall F ST distribution were considered as outliers, after which a false discovery rate correction of 0.05 was applied ( Supplementary Data 2 ). To examine the outlier F ST distribution compared with what would be expected from stochastic processes, we permuted the original dataset into 100 random replicates of two populations with 21 individuals each and plotted the outlier F ST distribution (means and 95% confidence intervals) against heterozygosity for all permuted population pairs. The outliers are in all but one case ( F ST =0.05) highly significantly above the random outlier F ST distribution. All of the 34 annotated genes could be assigned open-reading frames using the OrfPredictor online software [47] (available at http://proteomics.ysu.edu/tools/OrfPredictor.html ), using the output of a BLASTx to NCBI’s nr database as supporting data. Based on these, all outlier SNPs were identified as synonymous, non-synonymous or untranslated ( Supplementary Data 2 ). An over-representation analysis was performed using ErmineJ [48] based on the gene ontology annotation of the transcriptome, using an F ST of 0.08 as a cut-off (based on the F ST outlier permutation data). Functional categories significantly enriched in high F ST SNPs were graphed using the online GO visualization software ReVIGO [49] . How to cite this article: De Wit, P. et al . Forensic genomics as a novel tool for identifying the causes of mass mortality events. Nat. Commun. 5:3652 doi: 10.1038/ncomms4652 (2014). Accession codes: DNA sequences have been deposited in the NCBI short read sequence archive (SRA) under the accession code SRP037568 . A text file listing all identified polymorphisms and individual genotypes at all loci is available on DRYAD ( http://datadryad.org ), doi:10.5061/dryad.2qs35 .